Structural phase transformations in metallic grain boundaries Structural transformations at interfaces are of profound fundamental interest as complex examples of phase transitions in low-dimensional systems. Despite decades of extensive research, no compelling evidence exists for structural transformations in high-angle grain boundaries in elemental systems. Here we show that the critical impediment to observations of such phase transformations in atomistic modelling has been rooted in inadequate simulation methodology. The proposed new methodology allows variations in atomic density inside the grain boundary and reveals multiple grain boundary phases with different atomic structures. Reversible first-order transformations between such phases are observed by varying temperature or injecting point defects into the boundary region. Owing to the presence of multiple metastable phases, grain boundaries can absorb significant amounts of point defects created inside the material by processes such as irradiation. We propose a novel mechanism of radiation damage healing in metals, which may guide further improvements in radiation resistance of metallic materials through grain boundary engineering. Phase transformations at interfaces in crystalline materials are of significant fundamental interest and practical importance due to their possible impact on the macroscopic mechanical, transport and thermal properties of polycrystals [1] , [2] . To date, the studies of interfacial phase transitions have been focused primarily on ‘complexions’ of intergranular thin films in ceramics [3] , [4] , [5] and pre-melting transitions in metallic alloys [6] . Little is known about grain boundary (GB) transformations in single-component metals apart from the recently found dislocation pairing transition in low-angle GBs composed of discrete dislocations [7] . Despite decades of research, no convincing experimental or simulation evidence exists for structural transformations in high-angle GBs. Direct experimental observations of interfacial phase transitions by high-resolution transmission electron microscopy (HRTEM) are extremely difficult [8] , [9] , [10] , and to date evidence for the possibility of GB transformations has been obtained by less direct experimental methods. For example, recent measurements of diffusion in the Cu Σ5(310) GB (Σ being the reciprocal density of coincident sites [1] ) revealed a marked change in the temperature dependence of the diffusivity at about 800–850 K [11] , [12] , suggesting a possible structural transformation in this boundary. However, the concurrent molecular dynamics (MD) simulations [11] did not detect any structural change other than gradual accumulation of disorder and eventually GB pre-melting at high temperatures. Owing to the difficulty of experimental observations, much of the current knowledge about GB structures has come from computer simulations. Most of the MD simulations conducted to date have employed periodic supercells that did not permit variations in atomic density in the GB core region, which are possible under experimental conditions. This unphysical constraint stabilizes one particular GB structure and prohibits transformations to other structures with different GB densities. This can explain why transformations in high-angle GBs have not been found in the previous simulation work. We proposed a more general simulation approach that facilitates variations in GB density allowing the boundary to assume the most thermodynamically favourable structure. This approach reveals the existence of multiple GB phases characterized by not only different structures but also different densities. This opens the door, for the first time, to direct observations of transitions between GB phases with different densities in atomistic simulations of metallic systems. GB structures at 0 K To demonstrate this new approach, we studied two representative high-angle, high-energy Σ5(210) and Σ5(310) symmetrical tilt GBs in several FCC metals with atomic interactions described by embedded-atom method (EAM) (ref. 13 ) potentials. The choice of the Σ5(310) GB was motivated by the recent diffusion measurements described above [11] , [12] . The long-accepted structure of these Σ5 boundaries is an array of kite-shaped structural units ( Fig. 1b ). This structure is easily obtained by joining two perfect crystallites along (210) or (310) planes and applying various grain translations followed by static relaxation. It has been suggested, however, that in order to sample all possible structures of a GB its density must be also varied by adding or removing atoms [14] , [15] , [16] , [17] , [18] , [19] . We applied an algorithm which finds equilibrium GB structures at 0 K by varying the GB density along with grain translations and static relaxation. In Fig. 1 , we plot the obtained energies of the Σ5 GBs in Cu versus the extra number of atoms relative to a perfect crystal plane. The minima in this plot correspond to three different equilibrium structures: (i) the normal kites b and d, (ii) split kites c and e having extra 2/5 of the (310) plane or 7/15 of the (210) plane, respectively; and (iii) filled kites f having extra 6/7 of the (210) plane. Different cross-sections of the simulation block containing these structures were tested as illustrated in the Supplementary Fig. S1 . 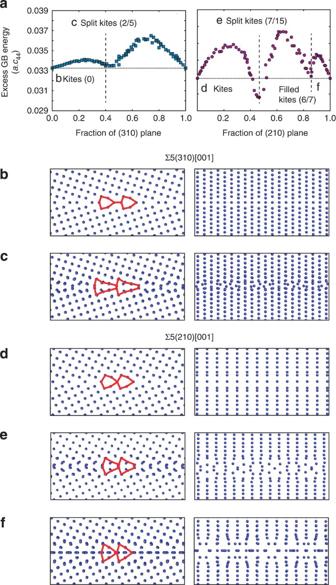Figure 1: GB structures and energies at 0 K. Results of structure and energy calculations for Σ5(310) and Σ5(210) GBs at 0 K using an EAM potential for Cu32. (a) GB energy versus atomic density (fraction of atomic plane) for the Σ5(310) (left) and Σ5(210) (right) GBs. The horizontal line marks the energy of the kite structure. The densities corresponding to local energy minima and the respective GB structures are indicated. Panels (b–f) show the GB structures as viewed parallel to the [001] tilt axis (left column) and normal to it (right column). (b,d) Normal kites. (c,e) Split kites. (f) Filled kites. Figure 1: GB structures and energies at 0 K. Results of structure and energy calculations for Σ5(310) and Σ5(210) GBs at 0 K using an EAM potential for Cu [32] . ( a ) GB energy versus atomic density (fraction of atomic plane) for the Σ5(310) (left) and Σ5(210) (right) GBs. The horizontal line marks the energy of the kite structure. The densities corresponding to local energy minima and the respective GB structures are indicated. Panels ( b – f ) show the GB structures as viewed parallel to the [001] tilt axis (left column) and normal to it (right column). ( b , d ) Normal kites. ( c , e ) Split kites. ( f ) Filled kites. Full size image For each structure corresponding to a local minimum of energy, we computed the excess GB energy [ U ] N , excess volume [ V ] N and two components of the GB stress, and , in the directions parallel and normal to the tilt axis, respectively [20] , [21] . The results summarized in Table 1 clearly demonstrate that the structures are characterized by significantly different thermodynamic parameters, including even different signs of the GB stress component . Table 1 Characteristics of different GB phases Full size table To demonstrate the generality of this important finding, similar calculations were performed with a different EAM Cu potential and for several other FCC metals including Ag, Au and Ni (see Supplementary Fig. S2 ). In all cases tested, the structures shown in Fig. 1 represented minima of the GB energy as a function of GB density. Remarkably, and contrary to the common belief, none of the tested potentials predicts the normal kites to be the lowest-energy structure of the Σ5(210) GB. The split kites are energetically more favourable for this boundary and are only slightly higher in energy than the normal kites for the Σ5(310) GB. GB-phase transformations with temperature The effect of temperature on the GB structures was studied by MD simulations with various boundary conditions starting with the normal-kite structure. First, we tested the traditional methodology with periodic boundary conditions. In the Cu Σ5(310) GB, the kites continued to exist up to ∼ 0.75 of the melting point T m =1,327 K. At higher temperatures the GB begins to disorder and eventually pre-melts near T m ( Fig. 2a ). This behaviour known from previous work [21] cannot explain the transformation suggested by the diffusion experiments [11] , [12] . A more complex behaviour was observed in the Σ5(210) GB. At about 400 K, the kites were found to transform into a structure similar to the filled kites (cf. Fig. 1f ). In Fig. 2b , a jump in thickness occurs between 300 and 400 K due to this change in GB structure. Similar behaviour was found in simulations with other EAM potentials for Cu, Au, Ag and Ni, suggesting that it represents a generic feature of FCC metals. However, these simulations impose a constraint on the supply of atoms into the GB core and do not reveal the full picture of possible structural changes. 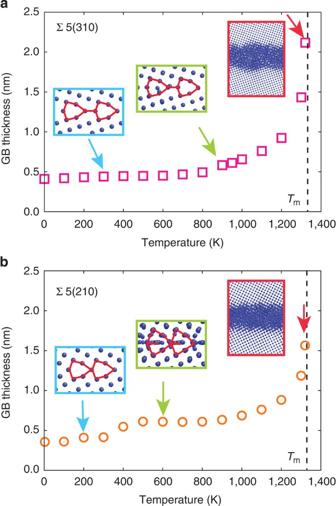Figure 2: MD simulations of GBs using periodic boundary conditions. The thickness of GBs at different temperatures was evaluated from the energy density profile across the GB. (a) The Σ5(310) GB gradually accumulates disorder and pre-melts near the melting pointTm, whereas (b) the Σ5(210) GB undergoes a transformation at 400 K before pre-melting nearTm. Figure 2: MD simulations of GBs using periodic boundary conditions. The thickness of GBs at different temperatures was evaluated from the energy density profile across the GB. ( a ) The Σ5(310) GB gradually accumulates disorder and pre-melts near the melting point T m , whereas ( b ) the Σ5(210) GB undergoes a transformation at 400 K before pre-melting near T m . Full size image For a more complete investigation, we modified the methodology by letting the GB terminate at an open surface as shown schematically in the Supplementary Fig. S3 . The surface serves as a source or sink of atoms, which may diffuse in or out of the GB to automatically adjust its density. The MD results are illustrated in Fig. 3 for an isothermal anneal at 800 K when the GB meets an open surface at one end and is constrained by a wall of fixed atoms at the other. In the simulation of the Σ5(310) GB initiated with the normal-kite structure, a new structure nucleates at the surface and grows inside the boundary. This structure can be identified as split kites, whereas the untransformed part of the boundary continues to be composed of normal kites. The extra atoms (40% of the (310) plane) required for the transformation are supplied by diffusion from the surface grove, a process that kinetically controls the transformation rate. Eventually, the new structure penetrates through the entire GB and reaches the fixed region. When the fixed atoms on the left are made dynamic (thus opening another surface), the entire GB reaches the transformed state ( Fig. 3e ). 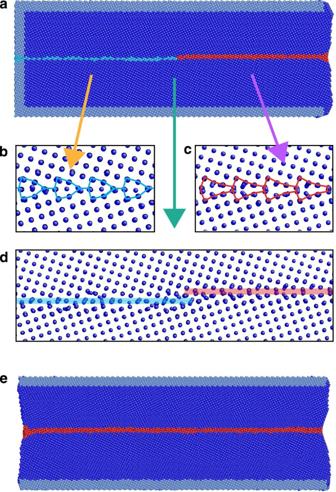Figure 3: High-temperature transformation of the Σ5(310) GB. (a) MD simulation of the Cu Σ5(310) GB at 800 K with an open surface allowing variations in GB density. The boundary undergoes a first-order phase transformation with the split-kite structure nucleating and growing from the surface. The normal-kite (b) and split-kite (c) structures are separated by a 1D-phase boundary accompanied by a step (d). (e) Completely transformed GB structure in the presence of two open surfaces. Figure 3: High-temperature transformation of the Σ5(310) GB. ( a ) MD simulation of the Cu Σ5(310) GB at 800 K with an open surface allowing variations in GB density. The boundary undergoes a first-order phase transformation with the split-kite structure nucleating and growing from the surface. The normal-kite ( b ) and split-kite ( c ) structures are separated by a 1D-phase boundary accompanied by a step ( d ). ( e ) Completely transformed GB structure in the presence of two open surfaces. Full size image The stability of the split-kite structure was tested by a series of isothermal anneals. It remained stable and well-ordered above 800 K and until ∼ 1,150 K when it began to disorder and pre-melt. Upon subsequent cooling from pre-melting temperatures to 1,000 K, the ordered split-kite structure reappeared inside the GB. This verifies the thermodynamic stability of the split-kite structure and eliminates any suspicion that its formation could be caused by the presence of the surface grove (an additional proof comes from the point-defect induced transformations in the absence of surfaces discussed below). We were unable to demonstrate the reversibility of the transformation back to normal kites by cooling the GB below 800 K because of the slow (on the MD time scale) diffusion rates at low temperatures. However, the zero-temperature results plotted in Fig. 1 establish that the normal-kite structure has the lowest energy and will be thermodynamically stable at sufficiently low temperatures. Figure 3d demonstrates that the two structures of the Σ5(310) GB can coexist and are separated by a line defect with an atomic-scale cross-section. This allows us to consider the two GB structures as two-dimensional (2D) phases separated a one-dimensional (1D) phase boundary. The phase transformation is first order and is kinetically controlled by GB diffusion. To our knowledge, this is the first observation of coexistence of two GB phases separated by a 1D-phase boundary in atomistic simulations. It is also evident that this phase boundary is associated with a GB step [22] . The exact nature of this 1D defect deserves a separate study in the future. As the two GB structures have different interface stresses and excess volumes, long-range elastic stresses could be generated around the 1D boundary between them. In principle, such stresses could affect the stability of the GB phases, for example, via the image forces arising due to the interaction of the stress field with boundary conditions. In our case, however, this effect was negligible due to the large size of the simulation block (about 12.5 nm in the y direction). For additional verification, simulations were repeated with different boundary conditions in the y direction and the same GB phases were invariably found. Similar transformations were found in the Σ5(210) GB in simulations starting from the filled-kite structure formed at 400 K. During isothermal anneals at temperatures below 1,050 K, the GB transforms into its thermodynamically stable phase at low temperatures: the split kites. This new phase grows from the surface and eventually penetrates through the entire boundary (cf. Fig. 4 ). When the boundary with split kites was heated up to 1,100 K, its structure transformed to filled kites ( Fig. 5 ). In this case, however, we were able to observe the reverse transformation. Upon subsequent cooling down to 1,000 K, the GB structure returned to the split kites, demonstrating full reversibility of the phase transformation. At temperatures close to T m this GB pre-melts by disordering of the filled-kite structure as observed earlier [23] . It is interesting to note that the normal-kite structure traditionally attributed to this boundary never appears as its thermodynamically stable phase. 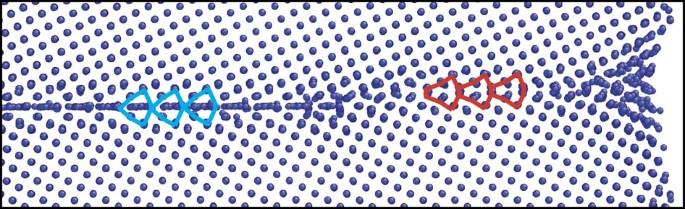Figure 4: High-temperature transformation of the Σ5(210) GB. MD simulation of the Cu Σ5(210) GB at 800 K with an open surface allowing variations in GB density. The boundary undergoes a first-order phase transformation from filled kites to split kites nucleating and growing from the surface. Figure 4: High-temperature transformation of the Σ5(210) GB. MD simulation of the Cu Σ5(210) GB at 800 K with an open surface allowing variations in GB density. The boundary undergoes a first-order phase transformation from filled kites to split kites nucleating and growing from the surface. 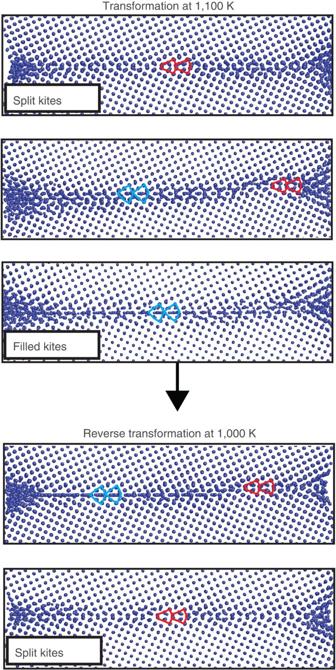Figure 5: Reversible GB-phase transformations induced by temperature. Σ5(210) GB terminated at two open surfaces. The initial split-kite structure taken from a prior anneal at 1,000 K transforms into filled kites at 1,100 K. Upon subsequent cooling and annealing at 1,000 K, it returns back to the split kites. Intermediate stages show the two GB structures: one growing from the surface and the other disappearing. It is concluded that the phase transition temperature is between 1,000 and 1,100 K. Full size image Figure 5: Reversible GB-phase transformations induced by temperature. Σ5(210) GB terminated at two open surfaces. The initial split-kite structure taken from a prior anneal at 1,000 K transforms into filled kites at 1,100 K. Upon subsequent cooling and annealing at 1,000 K, it returns back to the split kites. Intermediate stages show the two GB structures: one growing from the surface and the other disappearing. It is concluded that the phase transition temperature is between 1,000 and 1,100 K. Full size image GB phase transformations caused by point defects During the phase transformations, the GB absorbs/ejects large amounts of atoms from/to the surface. These absorption/ejection processes may have important implications for properties of polycrystals under extreme conditions. For example, in metals subject to radiation by energetic particles, large numbers of vacancies and interstitials are formed [24] . Interstitials are much more mobile than vacancies and reach sinks first, whereas the remaining vacancies can form clusters, stacking-fault tetrahedra and other defect complexes degrading the material properties. GBs can act as effective sinks of radiation-induced defects and can have a role in the damage healing. Some of the mechanisms of defect-GB interactions have been studied by MD simulations [25] , [26] . Our work suggests that the absorption of point defects can strongly modify the GB structure, causing structural transformations, which, in turn, can greatly increase the absorption capacity of the boundary. The proposed effect is illustrated in Fig. 6 . The simulation was intentionally performed in a periodic simulation block to exclude all sources/sinks of atoms other than the GB. The GB tested is Cu Σ5(310) and its initial structure consists of normal kites. This structure remains unchanged during anneals when no atoms are added to or removed from the system. We then introduce 80 interstitials into the GB region, which is equivalent to 40% of a (310) atomic plane. This fraction of the plane matches the local minimum of the GB energy corresponding to the split-kite structure (cf. Fig. 1a ). Upon anneal at 800 K, the interstitials diffuse into the GB core and get absorbed in it initially creating a disordered structure. As the anneal continues, the GB eventually orders into the split-kite phase. To demonstrate the reversibility of this radiation-induced transition, we then randomly remove the same number of atoms from the GB region, which simulates the insertion of radiation-produced vacancies. After a period of disorder, the GB structure transforms back to the normal kites. Thus, in the end of this phase transformation cycle the boundary returns to its initial state having annihilated a large amount of radiation-induced defects. A similar transformation cycle induced by absorption of point defects was observed in the Σ5(210) GB ( Supplementary Fig. S4 ). 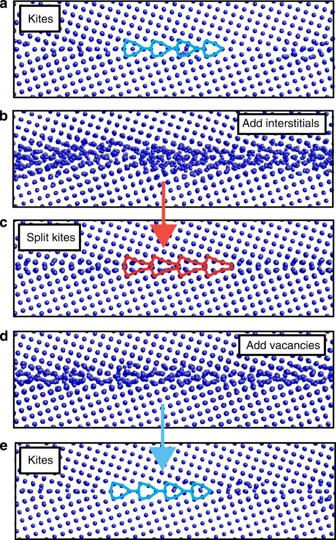Figure 6: Isothermal reversible GB-phase transformations induced by point defects. GB-phase transformations in the Cu Σ5(310) GB induced by interstitials and vacancies in a simulation block with periodic boundary conditions atT=800 K. After 80 interstitials are introduced into a 10 Å thick layer containing the GB, it transforms from the initial normal-kite structure (a) to a disordered state (b) and then to split kites (c). After the subsequent introduction of 80 vacancies into the same GB layer, the split-kite structure disorders (d) and then transforms back to normal kites (e). The GB states (a) and (e) are identical confirming that the transformation is fully reversible. Figure 6: Isothermal reversible GB-phase transformations induced by point defects. GB-phase transformations in the Cu Σ5(310) GB induced by interstitials and vacancies in a simulation block with periodic boundary conditions at T =800 K. After 80 interstitials are introduced into a 10 Å thick layer containing the GB, it transforms from the initial normal-kite structure ( a ) to a disordered state ( b ) and then to split kites ( c ). After the subsequent introduction of 80 vacancies into the same GB layer, the split-kite structure disorders ( d ) and then transforms back to normal kites ( e ). The GB states ( a ) and ( e ) are identical confirming that the transformation is fully reversible. Full size image Simulations of GB diffusion As discussed above, experimental measurements of GB diffusion in Cu bicrystals containing the Σ5(310) GB have been made by Budke et al . [12] and more recently by Divinsky et al [11] . The measurements revealed a marked change in the slope of the Arrhenius plot of the diffusivity at about 800–850 K [12] , [11] . To test the prediction that this change is caused by a structural phase transformation in this boundary, we performed MD simulations of the GB diffusivity using the methodology proposed in our previous work [27] , [28] , [29] . The simulations were performed separately for the normal-kite and split-kite structures. Recall that the normal kites are stable at low temperatures and transform to split kites at temperatures 800 K and higher. The results of the diffusion calculations are shown on the Arrhenius diagram in Fig. 7 . Note that the two GB structures have different diffusivities as well as activation energies. Furthermore, it is observed that the high-temperature split-kite phase has a lower activation energy (smaller slope) than the low-temperature normal-kite phase (larger slope). This trend closely correlates with the experimental measurements [12] , [11] , as does the approximate temperature at which the change in the slope of the Arrhenius diagram is expected. This agreement strongly suggests that the change in the GB diffusivity measured in the experiments [11] , [12] was caused by the phase transformation in this boundary. Further details of the diffusion simulations will be published elsewhere. 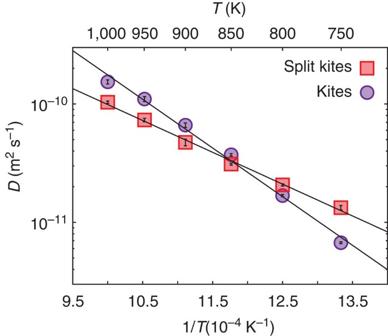Figure 7: Diffusivities of different GB phases Arrhenius diagram of the diffusion coefficient (D) calculated for two structures of the Σ5(310) boundary in Cu. Note the difference in the activation energy between the two GB structures. Figure 7: Diffusivities of different GB phases Arrhenius diagram of the diffusion coefficient ( D ) calculated for two structures of the Σ5(310) boundary in Cu. Note the difference in the activation energy between the two GB structures. Full size image In this work, we demostrate by atomistic simulations that high-angle metallic GBs can have multiple stable or metastable phases with different atomic structures and first-order transitions between them. For the particular symmetrical tilt Σ5 GBs studied here, we found three different phases. The normal-kite structure predicted to be the 0 K ground state of the Σ5(310) GB is consistent with room-temperature HRTEM observations [9] . The remaining two structures have not been seen by HRTEM yet but could have manifested themselves through sudden changes in temperature dependencies of GB properties such as diffusivity [11] , [12] . In fact, our simulations have shown that the GB phases found here are indeed characterized by different GB diffusion coefficients and that the slopes of their Arrhenius plots correlate with the experiment [11] , [12] . It should be recognized, however, that the present diffusion calculations can be compared with the experiment [11] , [12] only in terms of trends but not quantitatively. Whereas our diffusion calculations were performed for Cu self-diffusion, the experimental measurements were conducted for impurity diffusion of Ag in Cu. The latter process is accompanied by segregation of the diffusing atoms, which may potentially enhance the effect of the structural transformations on GB diffusion or even alter the GB phases and/or their transformation temperatures. The potential effects of solute segregation lie outside the scope of this paper. All three GB phases found in this work were reproduced in several FCC metals modelled with different atomistic potentials, suggesting that they represent a generic feature of FCC crystals. More general GBs may feature a larger variety of phases. The existence of GB phases in metals is likely to be a common phenomenon, which was previously overlooked owing to the overly constrained computer simulation methodology and challanges inherent in experimental atomic-level observations of GB structures at elevated temperatures. The finding of first-order transitions in elemental high-angle GBs is important as it provides a new testing ground for fundamental theories of GB thermodynamics and GB-phase transitions [30] . Future calculations of the exact transformation temperatures, transformation enthalpies as well as the excess thermodynamics properties of the 1D-phase boundaries would be of significant fundamental interest. In the future, this study could be extended to multicomponent systems that may additionally exhibit segregation-induced structural transformations with rather complex phase diagrams. In addition to the fundamental questions raised by this work, the present simulations suggest a possible novel mechanism of radiation damage healing in which a GB absorbs large amounts of point defects by transformation between different phases. It is believed that the same mechanism of defect absorption can operate under other extreme conditions involving high non-equilibrium concentrations of point defects, such as severe plastic deformation, diffusional creep and rapid grain growth in nano-crystalline materials. GB structure calculations at 0 K For each boundary, its energy was minimized for several different cross-sections of the periodic simulation block. A cross-section is defined by n × m , where n and m are the numbers of lattice periods in the directions parallel and normal to the tilt axis, respectively. For the Σ5(210) GB, we used the following cross-sections: 4 × 2, 6 × 1, 2 × 1, 7 × 2, 9 × 2, 11 × 2, 13 × 2 and 15 × 2. For the Σ5(310) GB, the cross-sections were 10 × 2, 8 × 2, 9 × 6, 9 × 2, 7 × 2 and 13 × 2. For each GB with a given cross-section, a number of trial configurations were generated and then minimized as follows, with the lowest minimized energy reported. First, relative translations of the two grains by vectors within a primitive cell of the displacement shift complete (DSC) lattice and all possible, non-equivalent, placements of the boundary plane in the direction normal to the boundary were generated. (These different placements are equivalent to relative translations by full DSC vectors). For example, for the 7 × 2 searches, 3 × 3 × 3 vectors within the DSC primitive cell were used, and the total number of configurations generated at this stage, including the different placements of the boundary plane, was 225. These will be referred to as base configurations below. For some searches more points within the DSC primitive cell were used. For each base configuration, all atoms within 15 Å of the nominal boundary plane were moved 0.001 Å in a (pseudo) random direction. Atoms that were very near each other were then removed to generate the configurations to be minimized. At each step of the removal process, the closest two atoms were both removed and an atom put back at the average position of the two that were removed. The process continued until no pair of atoms was within about 1/3 of the nearest neighbour distance. This was the first trial configuration to be minimized. After that, one atom was removed at a time (from the non-minimized configuration) to generate a configuration to be minimized. This was done until no pair of atoms was within about 0.99 of the nearest neighbour distance. In total, about 16,500 configurations were minimized in a 7 × 2 search for the Σ5(310) GB and about 24,000 for the Σ5(210) GB. The total number N of atoms removed could be larger than the number N 0 of atoms in a perfect plane parallel to the GB. In such cases, the GB density was determined by dividing N by N 0 and expressing the remainder as a fraction of N 0 . MD simulations at finite temperatures The MD simulations were performed in the canonical (NVT) ensemble with a Nosé–Hoover thermostat implemented in the ITAP molecular dynamics program [31] . The two symmetrical tilt GBs, Σ5(310)[001] and Σ5(210)[001], were created by joining two crystals rotated relative to each other around the [001] direction by the angle of 36.87° and 53.13°, respectively. The [001] tilt axis of the GB was aligned parallel to the x direction with the GB normal parallel to the y direction ( Supplementary Fig. S3 ). The system typically contained 150,000 to 250,000 atoms. Smaller blocks, containing about 50,000 atoms with periodic boundary conditions parallel to the GB plane, were used to compute the GB thickness, observe the GB pre-melting and simulate the GB transformations induced by vacancies and interstitials. In the simulations involving large blocks, the periodic boundary condition was kept in the x direction, whereas in the z direction the GB terminated at an open surface on one side and at a layer of fixed atoms on the other side. In some simulations, the GB terminated at open surfaces on both sides. The isothermal anneals of the GBs were performed at temperatures from 0 K to 0.98 T m . The boundary conditions were either fully periodic in the directions parallel to the GB plane or non-periodic when the GB was terminated at an open surface ( Supplementary Fig. S3 ). Additional simulations were conducted for the following FCC metals modelled with EAM potentials: Cu [32] , [33] , Ag [34] , Au [35] and Ni [36] . The GB atomic density changes were evaluated by comparing the number of atoms in a simulation block containing a given GB with the number of atoms in the initial block of the same cross-section containing an integer number of complete atomic planes. Relaxed GB structures were used to calculate the excess GB properties such as GB energy, volume and stress [20] , [21] . The calculations of the GB diffusion coefficients employed the methodology that was described in detail in previous work [27] , [28] , [29] and will not be repeated here. MD simulations of GB transformations induced by point defects In such simulations, the GB initially had the normal-kite structure, which was first annealed at 800 K for several nanoseconds. Then, 80 and 132 interstitials were randomly introduced inside a 1-nm thick layer containing the Σ5(310) and Σ5(210) GBs, respectively. These numbers of atoms correspond to 40% and 50% of the (310) and (210) planes, respectively. After the atoms were inserted, the isothermal anneal was continued at 800 K. The initial kite (respectively, filled-kite) structures quickly disappeared and significant atomic rearrangements took place in the boundary layer. However, within 1 to 100 ps of the simulation time the boundaries re-ordered into the split-kite structure. The obtained split-kite structures of both GBs were then taken as initial states to introduce vacancies in order to demonstrate transformations into metastable phases. The vacancies were introduced by randomly removing atoms within a 1-nm thick layer containing the GB. The number of vacancies was equal to the number of interstitials introduced previously. After 1 to 100 ps of the isothermal anneal at 800 K and a period of disorder, we observed a transformation into the normal-kite structure in the Σ5(310) GB and the filled-kite structure in the Σ5(210) GB. How to cite this article: Frolov, T. et al . Structural phase transformations in metallic grain boundaries. Nat. Commun. 4:1899 doi: 10.1038/ncomms2919 (2013).